Interface-induced nonswitchable domains in ferroelectric thin films Engineering domains in ferroelectric thin films is crucial for realizing technological applications including non-volatile data storage and solar energy harvesting. Size and shape of domains strongly depend on the electrical and mechanical boundary conditions. Here we report the origin of nonswitchable polarization under external bias that leads to energetically unfavourable head-to-head domain walls in as-grown epitaxial PbZr 0.2 Ti 0.8 O 3 thin films. By mapping electrostatic potentials and electric fields using off-axis electron holography and electron-beam-induced current with in situ electrical biasing in a transmission electron microscope, we show that electronic band bending across film/substrate interfaces locks local polarization direction and further produces unidirectional biasing fields, inducing nonswitchable domains near the interface. Presence of oxygen vacancies near the film surface, as revealed by electron-energy loss spectroscopy, stabilizes the charged domain walls. The formation of charged domain walls and nonswitchable domains reported in this study can be an origin for imprint and retention loss in ferroelectric thin films. One method of realizing a non-volatile logic element [1] is to use a ferroelectric material to induce a charge-mediated change of state in an adjacent material. A ferroelectric has a spontaneous electrical polarization that is switchable upon the application of a DC voltage [2] , [3] . However, a major issue for commercialization has been the poor reliability of ferroelectric memory devices including a decrease in polarization with repeated switching (fatigue), polarization backswitching leading to loss of data (retention loss) and preferential polarization state (imprint) [3] , [4] , [5] , [6] , [7] . Ground-state domain structures and switching processes in ferroelectric thin films are difficult to predict because of the importance of electrical and mechanical boundary conditions present at the film interfaces [8] . The primary mechanical boundary condition for an epitaxial thin film is the strain that results from the lattice mismatch between the film and substrate [8] , [9] , [10] , [11] . Electrical boundary conditions can dramatically influence ground-state domain structures and switching via polarization charge compensation mechanisms at the interfaces [12] , [13] , the formation of 180° stripe domains [14] , flux-closure domain structures [15] , [16] and interfacial reconstructions [17] . Mobile charge carriers arising from vacancies and impurities also play an important role by internally compensating the polarization charges or by modifying the electric field within the ferroelectric in response to an external bias [17] , [18] , [19] , [20] . In addition, achieving chemical potential equilibrium between ferroelectric thin films and electrode materials can cause the accumulation or depletion of mobile charge carriers, thereby leading to built-in potentials at the interfaces [18] , [19] , [21] . The macroscopic ferroelectric domain structures and their switching properties can be understood by directly visualizing domains during switching and characterizing the electrostatic potentials. Here, we report the unusual formation of charged 180° domain walls in head-to-head configuration in ferroelectric epitaxial thin films observed by dark-field transmission electron microscopy (TEM) combined with in situ electrical biasing [22] , [23] , [24] , [25] , [26] . Electrostatic potential and electric field distributions within ferroelectric films under external biases were, for the first time in our knowledge, mapped out using two techniques: off-axis electron holography [27] and electron-beam-induced current (EBIC) measurement [28] . We found that electronic band bending across the film/substrate interfaces pins the local polarization direction and produces unidirectional biasing fields, inhibiting local domain switching and leading to formation of charged 180° domain walls in an unstable head-to-head configuration. Surprisingly, these positively charged domain walls were found to be stable over several months. Our electron-energy loss spectroscopy data revealed higher concentration of oxygen vacancies near the film surface, which implies internal charge compensation by mobile charge carriers. Characterization of domain structures Epitaxial PbZr 0.2 Ti 0.8 O 3 (001) (PZT) thin films were grown on 0.5 wt.% Nb-doped SrTiO 3 (001) (Nb-STO) by off-axis radiofrequency magnetron sputtering at 515 °C and cooled to room temperature in 225 mTorr of process gases. To facilitate in situ electrical biasing of the PZT films, a capacitor geometry with conventional Pt electrodes is fabricated using focused-ion beam (FIB) after Au sputtering, as shown in Fig. 1a (ref. 27 ). A probe electrical contact in the TEM holder (Nanofactory Instruments AB) is made to the top electrode in situ in TEM, while the counter electrode is connected to the conducting Nb-STO substrate using silver paste. To maximize contrast associated with 180° ferroelectric domains because of violation of Friedel’s law [29] , [30] , samples were tilted from the [010] zone axis for a two-beam condition and dark-field images were obtained with series of external biases ( Figs 1a and 2a–e ). Owing to ~1.2% biaxial compressive strain, the PZT thin films consist primarily of domains with out-of-plane polarization [31] , although they are likely fully relaxed because of the presence of misfit dislocations near the interface. The c domains in as-grown PZT thin films have the polarization direction, either upwards or downwards, which are henceforth referred to as P up or P down domains, respectively. Conventionally, stripe patterns with alternating polarization direction have been predicted theoretically as a ground domain structure and experimentally observed for ferroelectric thin films [1] . However, we observed the domain structure in as-grown PZT film shown in Fig. 1c showing surprisingly two domains with opposite polarizations met in the middle of a film in a head-to-head configuration. Previously, occurrence of charged domain walls, especially during polarization-switching process, has been reported from various in situ switching experiments [22] , [23] , [24] , [32] . However, the head-to-head domain structure observed in the as-grown PZT thin films is remarkable as such domain walls are positively charged and thus energetically unfavourable for a ground state. Furthermore, domain walls are not flat, but rather zigzag in shape, with an additional energy cost associated with this configuration. The zigzag-like domain walls can be a consequence of domain wall pinning at structural defects within the film [33] . Piezoresponse force microscopy (PFM) result ( Fig. 1d ) also supports the presence of charged domain walls embedded in PZT thin films showing an intermediate piezoresponse signal for an as-grown region compared with two oppositely poled regions with ±10 V. Note that stripe domains with alternating 180° domains can be ruled out by the monotonous contrast in the PFM image. A typical current–voltage ( I–V ) curve ( Fig. 1b ) taken from the TEM sample in Fig. 1a shows a rectifying property of Au top electrode/PZT/Nb-STO structure. Similar electric transport properties have been reported for PZT films grown on Nb-STO substrates, attributed to pn junction-like band bending at the film/substrate interface [34] . We notice two paths of leakage currents for TEM samples prepared by FIB milling. The first contribution is from mobile charge carriers in ferroelectric films because of vacancies and impurities serving as dopants and defect-mediated conduction such as Frenkel-Poole conduction considering large concentration of structural defects associated with strain relaxation [3] . The second is from FIB-milling-induced damages on the top and bottom surfaces of cross-sectioned TEM samples [27] . The latter can be minimized by careful FIB milling with low-energy Ga + ions. These leakage currents can be approximated as a linear resistor connected in parallel to the ferroelectric films. However, the clear rectifying behaviour shown in Fig. 1b suggests that charge transport is not controlled by the leakage. We also point out that illuminating the PZT/Nb-STO interface with the TEM electron beam generates excess charge carriers and thus increases conductivity of the film similar to optical excitations. With illumination of 200 kV electron beam at a beam current of ~1 nA, additional currents are measured for both positive and negative biases, as shown in Fig. 1b . A small open-circuit voltage ( V OC ) of −0.4 eV is measured under electron beam illumination, as shown in the inset of Fig. 1b . 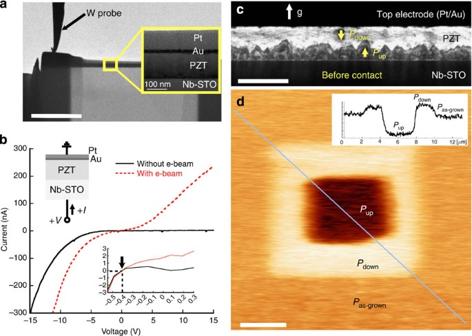Figure 1: Epitaxial PZT thin films on Nb-STO substrate. (a) A TEM image showing an electrical contact made forin situbiasing experiment. The scale bar is 2 μm. (b) A typical current–voltage (I–V) curve from the TEM sample showing a clear rectifying behaviour. The insetI–Vshows −0.4 V ofVOC. (c) A DF TEM image with the 003 reflection of PZT lattice showing unusual head-to-head charged domain walls formed in the as-grown PZT film. The scale bar is 200 nm. This image was taken before making an electrical contact. (d) A PFM image containing two oppositely poled states (dark contrastPupand bright contrastPdown) with external biases of 10 V in magnitude. The scale bar is 2 μm. Background is the as-grown state. Figure 1: Epitaxial PZT thin films on Nb-STO substrate. ( a ) A TEM image showing an electrical contact made for in situ biasing experiment. The scale bar is 2 μm. ( b ) A typical current–voltage ( I–V ) curve from the TEM sample showing a clear rectifying behaviour. The inset I–V shows −0.4 V of V OC . ( c ) A DF TEM image with the 003 reflection of PZT lattice showing unusual head-to-head charged domain walls formed in the as-grown PZT film. The scale bar is 200 nm. This image was taken before making an electrical contact. ( d ) A PFM image containing two oppositely poled states (dark contrast P up and bright contrast P down ) with external biases of 10 V in magnitude. The scale bar is 2 μm. Background is the as-grown state. 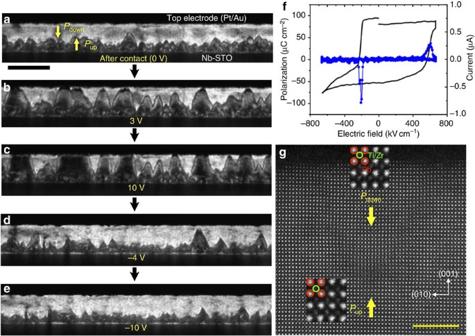Figure 2: Domain switching behaviour. (a–e) A series of DF TEM images showing domain-switching behaviour induced by a series of external biases. The scale bar is 200 nm. Sequence of biasing is shown with arrows. The 0-V image (a) was taken right after making the electrical contact, which shows similar domain structure asFig 1c. Note that domain switching do not occur near the bottom interface. (f) AP-Eloop obtained from PZT thin film with switching currents (blue). (g) An atomic resolution STEM-HAADF image of a head-to-head domain configuration. The scale bar is 5 nm. Two insets are enlarged images for each domain showing that the Ti/Zr columns are displaced upwards (downwards) with respect to the Pb columns for thePdown(Pup) domain. Yellow arrows indicate the polarization directions. Full size image Figure 2: Domain switching behaviour. ( a – e ) A series of DF TEM images showing domain-switching behaviour induced by a series of external biases. The scale bar is 200 nm. Sequence of biasing is shown with arrows. The 0-V image ( a ) was taken right after making the electrical contact, which shows similar domain structure as Fig 1c . Note that domain switching do not occur near the bottom interface. ( f ) A P-E loop obtained from PZT thin film with switching currents (blue). ( g ) An atomic resolution STEM-HAADF image of a head-to-head domain configuration. The scale bar is 5 nm. Two insets are enlarged images for each domain showing that the Ti/Zr columns are displaced upwards (downwards) with respect to the Pb columns for the P down ( P up ) domain. Yellow arrows indicate the polarization directions. Full size image In situ domain switching The domain evolution under various external biases using dark-field TEM imaging combined with in situ electrical biasing is summarized in Fig. 2 . Upon application of positive bias, P up domains (dark region) grow towards the top interface. With 3-V bias, some P up domains reached the top electrode but significant areas near the top electrode are left unswitched, indicating that domain switching is highly inhomogeneous, possibly because of random domain wall pinning by structural defects. Under a negative applied bias, P down domains (bright region) grow towards the bottom interface. However, in this case, no P down domain reaches the bottom interface, resulting in the formation of charged 180 o domain walls in the film. Application of negative bias up to −15 V (not shown here) does not result in domain switching beyond that shown in Fig. 2e . It can be concluded that switching behaviour observed in Fig. 2 is highly asymmetric ( P up domain is preferred) and P up domain near the bottom interface is not switchable. A P-E loop obtained from PZT thin films also shows an asymmetric switching, as shown in Fig. 2f . Here the electric fields are estimated with the PZT film thickness of 150 nm. The remnant polarizations are about 80 and 50 μC cm −2 for P up and P down domains, respectively. We find that this P-E loop agrees well with the TEM observations in Fig. 2a–e . The negative switching current sharply peaked near −0.2 MV cm −1 agrees with rapid switching at −4 V ( Fig. 2d ) followed by almost no additional switching with −10 V ( Fig. 2e ). For the positive switching, a dramatic switching occurs between 0 and 3 V ( Fig. 2b ) and switching continues between 3 V ( Fig. 2b ) and 10 V ( Fig. 2c ) without completing switching, implying that the coercive field for P up switching is not sharply defined but rather broadly ranged around 10 V (~0.67 MV cm −1 ), in agreement with the P-E loop. To ensure that the contrasts observed in dark-field TEM images are indeed 180 o head-to-head domains, we obtained atomic resolution high-angle annular dark-field (HAADF) scanning TEM (STEM) images after further thinning the TEM sample using low-energy (900 eV) Ar-ion milling. As shown in Fig. 2g, a triangular domain is clearly visible and the Ti/Zr columns are displaced in the opposite direction along the c axis across the domain wall. For Ti-rich PZT thin films, the polarization direction is antiparallel with the Ti/Zr displacement direction with respect to the Pb latttice [13] , [16] . We attribute the development of triangular domain shapes to anisotropy of domain growth [3] . Considering two components of domain wall speed for a given electric field, v a and v c , along the a axis and c axis, respectively, we estimate that ν c is approximately two to three times faster than ν a based on the domain shapes in Fig. 2 . It should be noted that both domain wall pinning by defects and anisotropic domain growth can be ruled out as an origin for the asymmetric domain switching and nonswitchable P up domains near the bottom interface. Especially, domain wall pinning can be easily overcome by applying a larger field. Recently, Gao et al . [24] reported that the pinning force of misfit dislocations on domain wall motion is rather weak and slows down domain wall speed slightly. The domain wall pinning at defects plays some important roles in domain switching. However, the focus of this study is on the origins of the asymmetric switching and the nonswitchable P up domains near the PZT/Nb-STO interface. Electric field mapping In order to understand the origin of the nonswitchable interface polarization, we have mapped out electrostatic potentials and electric field distributions in PZT thin films under biased conditions using two different techniques: off-axis electron holography ( Fig. 3 ) and EBIC measurements ( Fig. 4 ). Electrostatic potential distributions were determined via electron-wave phase retrieval with various external biases, as shown in Fig. 3a–c . Electric potentials in the Nb-STO substrate increases with +15 V compared with that in PZT film and vice versa for −15 V, clearly showing local potential changes because of application of external biases. However, any potential changes associated with the charged domain walls or depolarization field within domain are not detected in the unbiased (0 V) phase map ( Fig. 3a ), possibly because of effective compensation of the polarization charges at domain walls by mobile charge carriers or insufficient phase sensitivity of electron holography. In addition, no significant built-in potential across the PZT/Nb-STO interface is observed in the reconstructed phase image under 0 V biasing. In our experiment, to avoid diffraction contrast related with dynamic variation of external biases resulted from the converse piezoelectric effect and non-uniform sample thickness, we extract the changes in electrostatic potential distributions solely caused by external biases by taking differences between the phase shifts obtained under external bias conditions and that under 0 V (see Methods section). The line profiles in Fig. 3d show a considerable deviation from a linear potential distribution that one would expect for a pure dielectric assumption where no mobile charge carriers are considered. Especially, a noticeable potential barrier develops at the PZT/Nb-STO interface and increases as the positive bias applied to Nb-STO is increased. In addition, distribution of electric fields along the c axis ( Fig. 3e ), obtained by taking the first derivative of potential line profiles ( Fig. 3d ), shows that the electric fields are concentrated near the PZT/Nb-STO interface under positive biases. Here the positive sign of the electric field points from the bottom electrode to the top electrode. When negative biases are applied to Nb-STO, nearly no potential barriers and potential slopes are found at the PZT/Nb-STO interface (blue lines in Fig. 3e ). This unidirectional bias field near the PZT/Nb-STO interface can yield only P up domains, not P down domains, because applying negative bias to the substrate generates insufficient fields to initiate domain switching from P up to P down . As a consequence, P up domains near the PZT/Nb-STO interface are unswitchable, in agreement with domain switching behaviour observed in Fig. 2 . 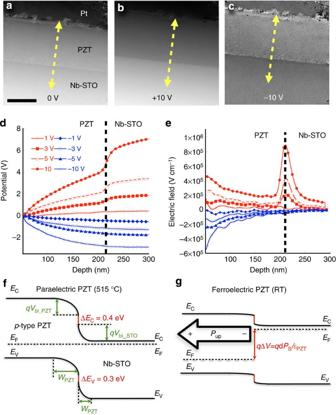Figure 3: Electrostatic potential and electric field mapping using off-axis electron holography. (a–c) Reconstructed phase images with external biases of 0 (a), +15 (b) and −15 V (c), respectively, taken on the same area of PZT thin film. The scale bar is 100 nm. (d,e) Line profiles of electrostatic potentials (d) and electric fields (e) quantified for the areas indicated ina–cwith arrows. Potentials and fields shown here were taken with respect to 0-V phase image (See Methods section). The potential at the Au/PZT interface has been chosen as a reference (0 V or electrical ground). (f,g) Schematics of band bending across PZT/Nb-STO in paraelectric (f) and ferroelectric states (g) of PZT films. Note that negative polarization charges near the interface suppress the band bending. Figure 3: Electrostatic potential and electric field mapping using off-axis electron holography. ( a – c ) Reconstructed phase images with external biases of 0 ( a ), +15 ( b ) and −15 V ( c ), respectively, taken on the same area of PZT thin film. The scale bar is 100 nm. ( d , e ) Line profiles of electrostatic potentials ( d ) and electric fields ( e ) quantified for the areas indicated in a – c with arrows. Potentials and fields shown here were taken with respect to 0-V phase image (See Methods section). The potential at the Au/PZT interface has been chosen as a reference (0 V or electrical ground). ( f , g ) Schematics of band bending across PZT/Nb-STO in paraelectric ( f ) and ferroelectric states ( g ) of PZT films. Note that negative polarization charges near the interface suppress the band bending. 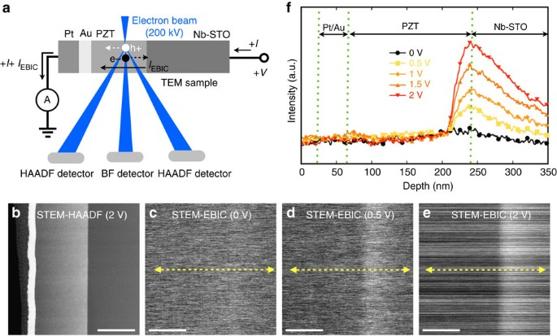Figure 4: Mapping electron-beam-induced current. (a) A schematic of simultaneous acquisition of STEM-HAADF and STEM-EBIC images. (b) A STEM-HAADF image taken with 2 V on Nb-STO substrate. (c–e) STEM-EBIC images taken with 0, 0.5 and 2 V, respectively.b,ewere acquired simultaneously. All scale bars are 50 nm. (f) Line profiles of STEM-EBIC signals from the areas indicated inc–e. Full size image Figure 4: Mapping electron-beam-induced current. ( a ) A schematic of simultaneous acquisition of STEM-HAADF and STEM-EBIC images. ( b ) A STEM-HAADF image taken with 2 V on Nb-STO substrate. ( c – e ) STEM-EBIC images taken with 0, 0.5 and 2 V, respectively. b , e were acquired simultaneously. All scale bars are 50 nm. ( f ) Line profiles of STEM-EBIC signals from the areas indicated in c – e . Full size image We also measured EBIC signals under various external biases to further investigate electric field distributions. Total electric currents flowing through the sample have been collected as an analogue signal for each electron-beam position during electron beam scanning with dwell time of 32 μs during the STEM-HAADF image acquisition, as shown in Fig. 4a . When a 200-keV-electron beam passes through the sample, it excites core level and valence electrons to conduction bands (CBs), generating electron–hole pairs (ehps). In the absence of electric field, these ehps diffuse out before they eventually recombine, yielding no net current. However, nonzero local electric fields can separate these ehps, generating an additional current ( I EBIC ). Since ehp separation occurs more effectively under higher electric fields, I EBIC is proportional to local electric field intensities smoothed by excess carrier diffusion. Previously, in the case of Si TEM samples, we have shown that the excess carrier diffusion length can be significantly reduced because of the enhanced surface recombinations [28] . We note that the EBIC signals collected with negative biases on Nb-STO were very noisy because of large forward currents flowing through the sample ( Fig. 1b ). Figure 4b–e shows a series of simultaneously acquired STEM-EBIC and STEM-HAADF images under various positive biases. Although EBIC images are noisy because of the dynamic scanning noise of the electron beam, we can clearly see a bright band developing near the PZT/Nb-STO interface with increasing positive applied biases. This bright band suggests that large electric fields are indeed induced at the heterojunction with positive biasing, agreeing with the electric fields mapped out by electron holography ( Fig. 3e ). Under zero bias, there is a small and broad EBIC signal near the interface suggesting nonzero electric field associated with the band bending across the interface. Interestingly, EBIC signals expand more rapidly in the Nb-STO side with increasing positive biases than in the PZT film. EBIC signals in PZT film are confined to ~40 nm near the interface and are independent of bias voltage. This behaviour is also observed in potential profiles ( Fig. 3d ) obtained by off-axis electron holography. We attribute this to the presence of a higher concentration of deep levels continuously distributed throughout the band gap of PZT film, especially near the heterojunction due to large amount of structural defects associated with the lattice mismatch at the interface. These deep levels are perhaps mostly acceptor-like and trap electrons. In addition, converse piezoelectric effect of the PZT film may induce additional polarization charges with increasing biases. The observed nonlinear potential profiles (that is, inhomogeneous electric fields) and unidirectional bias fields, consistently observed by both off-axis electron holography and EBIC measurements, can be explained if we consider PZT and Nb-STO as wide band gap semiconductors that have electronic band bending across the heterojunction. According to the electron affinity rule, there is a type II band alignment across the PZT/Nb-STO heterojunction with 0.4 eV CB offset and 0.3 eV valence band offset [35] , as shown in Fig. 3f . The electron concentration in 0.5 wt% Nb-doped STO is ~2.2 × 10 20 cm −3 , which pushes the Fermi level of Nb-STO close to the edge of the CB edge [36] . The PZT film behaves as a highly compensated semiconductor because of Pb and O vacancies, as well as deep levels associated with large amounts of structural defects because of the lattice mismatch [37] , [38] . In this work, we assume PZT is a p -type conductor with effective dopant concentration ( N eff ) of ~10 20 cm −3 considering acceptor-type deep levels and shallow doping levels [39] . Without considering local polarization charges, 1.9-V built-in potential is drawn for the heterojunction between PZT thin film and Nb-STO substrate, as shown in Fig. 3f . According to the heterojunction band alignment theory [40] , the potential drops ( V PZT and V STO ) and depletion region widths ( W PZT and W STO ) supported by each PZT and Nb-STO under thermal equilibrium and the depletion approximation can be determined as: where V bi is the built-in potential, ε PZT and ε STO dielectric constants for PZT and Nb-STO, respectively, N D dopant concentration in Nb-STO, q electronic charge and V reverse bias. An estimate of each built-in potentials and depletion regions can be made if the dielectric constants of PZT and Nb-STO are known. Inserting ε PZT =200 ε 0 (ref. 39 ) and ε STO =50 ε 0 (ref. 41 ) into the above equations gives V bi_PZT =0.67 V and V bi_STO =1.23 V, and W PZT =12 nm and W STO =6 nm, respectively, under zero bias. The charge neutrality condition is met by qW PZT N eff = qW STO N D ~19.2 μC cm −2 . The PZT/Nb-STO heterojunction is therefore expected to exhibit a rectifying property since positive bias or negative bias applied to Nb-STO will increase or decrease, respectively, the energy barrier for an electron injection from the Nb-STO. Under reverse (positive) bias, most of the applied voltage is drawn across the reverse-biased PZT/Nb-STO, while under forward (negative) bias, negligibly small voltage across the forward-biased PZT/Nb-STO, being consistent with electron holography ( Fig. 3 ) and EBIC results ( Fig. 4 ). Linear potential profiles near the top interface for both positive and negative biases in Fig. 3 suggest Ohmic-like behaviour of the top interface. This Ohmic behaviour can be attributed to high density of interface states due to extended exposure of PZT film surface to atmosphere after film deposition and room-temperature top electrode (Au) deposition. Conduction across the top electrode/PZT interface occurs through these interface states, not by band bending. As a consequence, electric transport is mainly governed by minority carrier (electron) injection across the PZT/Nb-STO interface, leading to a rectifying behaviour. The polarization charge near the interface will influence the zero-bias band bending and the associated built-in potential. Conceptually, polarization charge can be treated as an equivalent to an external bias to induce the same amount of charge within the PZT film [42] . The presence of negative polarization charge of P up domain near the PZT/Nb-STO interface can be considered as a forward biasing the heterojunction (negative bias to Nb-STO), inducing the same amount of charge as the spontaneous polarization ( P S ). Consequently, the negative polarization charge of the P up domain counteracts total space charges on both sides of the heterojunction. The sum of total space charge densities stored in both depletion regions in the band diagram shown in Fig. 3f under zero bias is 38.4 μC cm −2 , which is comparable to typical polarization charges reported for epitaxial PZT thin films. Another simple way to estimate influence of polarization charges on band bending is using the dielectric gap model [39] that considers polarization charge as a sheet charge separated from the interface by a dielectric gap to give rise to a change in built-in potential, . Here Δ V is a change in built-in potential because of presence of polarization charge located from the heterojunction by a gap ( d ). Estimation of Δ V requires knowledge of exact values of P S , ε PZT and d . For an epitaxial PZT film, it is reported that the band bending modulation because of polarization charge can be of the order of 0.71 eV [43] using 150 as the PZT dielectric permittivity, 1 nm gap and 95 μC cm −2 of polarization charge. We note that the dielectric constant in the gap within the PZT film near the interface can be significantly lower than that of intrinsic PZT. This would significantly increase the band bending modulation. Interestingly, a dielectric permittivity of ~50 for the gap layer results in a flat band condition across the PZT/Nb-STO heterojunction (exactly cancelling out the built-in potential of 1.9 eV) if we assume 80 μC cm −2 polarization charge for PZT film and 1-nm dielectric gap. This ‘flat-band’ scenario ( Fig. 3g ) is supported by off-axis electron holography and EBIC data that show no measurable band bending or small I EBIC across the PZT/Nb-STO interface under zero-bias condition, as shown in Figs 3 and 4 . Origin of the charged domain wall formation One scenario leading to the formation of head-to-head domain walls in as-grown PZT thin films is as follows. We assume that the PZT films were grown in the paraelectric phase because of the high deposition temperature of 515 °C. Owing to the band bending across the PZT/Nb-STO heterojunction, a built-in electric field pointing from Nb-STO to PZT will be induced within the depletion region. When the PZT film goes through the paraelectric–ferroelectric phase transition upon cooling, the P up domain will be induced near the interface because its polarization direction is parallel to the built-in electric field within the PZT depletion region. However, near the surface of the PZT film depending on local chemistry and defect natures, opposite built-in electric field can be present. We investigated local Ti valence changes in the PZT thin films using electron-energy loss spectroscopy (EELS). 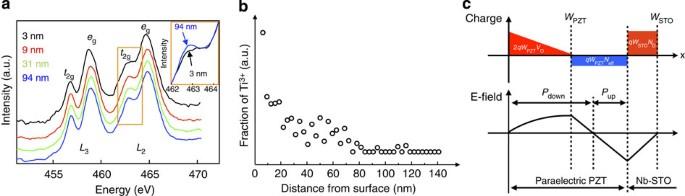Figure 5: Progress transition of Ti valence states. (a) EELS spectra of Ti-L edges for different positions in PZT film. A 2D spectrum image (22 × 63 pixels) was acquired with 3.1 nm pixel width from a rectangular region. Lateral (in plane direction) 22 spectra were summed to enhance signal-to-noise ratio. Each number indicates the distance in nm from the surface of the PZT film. (b) Multiple least-square fitting results with the 94 nm spectrum as a reference. (c) A schematic of charge (top) and electric field (bottom) distributions in paraelectric PZT film.VOrepresents the concentration of doubly charged oxygen vacancy. Figure 5a shows a series of Ti-L edges from several positions in the PZT film as a function of distance from the top interface. A systematic trend, especially regarding the change of the Ti L 2 peak intensities, is observed when comparing with the Ti L 2 edge taken from 94 nm away from the top interface. The Ti L 2 edge taken near the top interface (3 nm away from the surface) shows two main constituent peaks ( t 2g and e g ) develop noticeable shoulders, as shown in the inset of Fig. 5a , in agreement with trends reported in the literature [44] . Using the Ti-L edge far from the surface (94 nm away) as a reference, we plotted the differences in Ti-L edges using a multiple least-square fitting ( Fig. 5b ). This shows a progressive transition in the relative Ti valence state towards the surface of the PZT film. Although the exact valence state of Ti at the surface is difficult to quantify, the subtle change of Ti valence suggests more conduction electrons near the surface of PZT film, implying the presence of oxygen vacancy in the PZT film. A higher concentration of oxygen vacancy near the surface of PZT film will generate a net electric field pointing from the surface to the film/substrate interface, inducing P down domains near the surface region of PZT, despite of the energy cost for the formation of head-to-head 180° domain walls. Mobile electrons from near-surface oxygen vacancies will migrate and accumulate around the charged domain walls for its stabilization via internal charge screening. Mokry et al . [45] reported in their theoretical study that free charge compensation of bound charge can lead to a strong reduction in the pressure exerted on charged domain wall from an external electric field. This supports the scenario described here, of bound charge compensation by mobile charge carriers for their stabilization. A schematic for charge distributions and built-in electric fields in paraelectric phase of the PZT film is shown in Fig. 5c . This scenario is similar to a back-to-back Schottky diode model for metal–ferroelectric–metal structures [39] , where two opposite built-in electric fields pointing at each other are set from the top and bottom electrode interfaces. Figure 5: Progress transition of Ti valence states. ( a ) EELS spectra of Ti-L edges for different positions in PZT film. A 2D spectrum image (22 × 63 pixels) was acquired with 3.1 nm pixel width from a rectangular region. Lateral (in plane direction) 22 spectra were summed to enhance signal-to-noise ratio. Each number indicates the distance in nm from the surface of the PZT film. ( b ) Multiple least-square fitting results with the 94 nm spectrum as a reference. ( c ) A schematic of charge (top) and electric field (bottom) distributions in paraelectric PZT film. V O represents the concentration of doubly charged oxygen vacancy. Full size image Our study reveals that the built-in electric fields associated with electronic band bending across the PZT/Nb-STO heterojunction and higher oxygen vacancy concentration near the surface of the PZT film induce P up and P down domains, respectively, upon paraelectric–ferroelectric phase transition, which counteract each built-in electric field. The heterojunction behaves as a pn junction and produces unidirectional bias fields, prohibiting domain switching of P up domains near the heterojunction. As a result, energetically unfavourable charged domain walls with head-to-head configuration are induced in the middle of PZT films during domain switching process initiated by external biasing. These charged domain walls are found to be stable because of internal charge compensation by mobile charge carriers in the PZT film. Our observation of nonswitchable P up domains near the PZT/Nb-STO interface and formation of charged domain walls in the middle of the PZT film can be an origin of imprint (preferred P up ( P down ) domains near the bottom (top) interface) and retention loss (possible backswitching near the top and bottom interfaces) in ferroelectric thin films. We also point out that the switchable diode effects have not been previously observed for PZT thin films [42] , in contrary to BiFeO 3 (ref. 46 ). Our results imply that a nonswitchable P up domain near the bottom interface can be the origin for the absence of band bending modulation by polarization charge in the PZT/Nb-STO system. Thin film growth and characterization Thin films of PZT are grown on 5 × 5 × 0.5 mm samples of 0.5 wt.% Nb-STO (001) obtained from Crystec. The films of PZT are grown using off-axis radiofrequency magnetron sputtering, under flowing Ar (33.7 sccm) and O 2 (13.7 sccm), where sccm refers to the cubic centimetres per minute at standard temperature and pressure. The chamber pressure is maintained at 225 mTorr and the substrate temperature is 515 °C. The deposition rate is calibrated using X-ray reflectivity and is ~4.5 Å min −1 . The samples are cooled in the process gases at a chamber pressure of 225 mTorr. The thickness of films analysed here are ~150 nm. X-ray diffraction scans ( Supplementary Fig. 1 ) demonstrate the growth of high-quality single crystalline films of PZT. The (001) rocking curve ( Supplementary Fig. 1c ) has a full-width half maximum of 0.04°, the same as the Nb-STO substrate. PFM PFM was performed by writing squares with a DC bias voltage of ±10 V. Readout was performed with an AC-excitation voltage of 1 V, at a frequency far off resonance. P-E loop measurement was performed with an aixACCT ferroelectric tester on a PZT thin film sample using a pulsed positive up negative down measurement (150 nm PZT on Nb-STO (001)). The pulsed measurement facilitates subtraction of the leakage current, leaving only the switching current. TEM Final FIB milling for TEM sample preparation was carried out using 5 keV Ga + ions to minimize ion-beam-induced damages. For STEM-HAADF, the sample was further milled with 900 eV Ar ions with ±10° incidence angles using Nanomill (Fischione Instruments Inc.). A JEOL 2100F Lorentz microscope was used for off-axis electron holography. A JEOL ARM 200CF equipped with a cold field-emission gun and double-spherical aberration correctors at the Brookhaven National Laboratory operated at 200 kV was used for STEM-HAADF. The collection angles for HAADF detectors were from 68 to 280 mrad. EBIC signals were acquired simultaneously with STEM-HAADF images with the preamplifier installed with holder controller provided by Nanofactory Instruments AB. EELS data were obtained with 0.1 eV/ch dispersion. Data analysis of electron holograms The electrostatic potential distributions across top electrode/PZT/Nb-STO under external biases were mapped out by off-axis electron holography. Phase shift φ ( x ) 0V in imaging 200 keV electron wave measured using electron holography under zero external bias condition is quantitatively related to electrostatic potentials within the sample and local thickness t ( x ) in (nm) as the following; where C E is a constant of 0.00729, rad V −1 ·nm for 200 keV electron beam, V MIP ( x ) the mean inner potential in (V) and V bi ( x ) the built-in potential in (V). Here the x axis is taken along the c axis and no fringing fields outside TEM samples are assumed. V MIP ( x ) is the mean inner potential that the imaging electron would see in the crystal and differs for PZT film and Nb-STO substrate. If we neglect unit-cell volume changes under biased conditions because of converse piezoelectric effects of PZT thin films, then V MIP ( x ) can be treated as a constant. V bi ( x ) is associated both with the depolarization fields because of uncompensated polarization charges in PZT thin films and the built-in electric fields across top and bottom interfaces because of electronic band bending to reach a electrochemical equilibrium. If we assume the full polarization charge compensation at the top interface, then V bi ( x ) across the PZT film is mainly attributed to the electronic band bending across the PZT/Nb-STO heterojunction as a result of charge exchange considering the effects of polarization charge. We estimate that V bi ( x ) at 0 V is small for P up domain in PZT film from EBIC ( Fig. 4 ) because the EBIC is proportional to charge collection volumes in the sample, that is, product of depletion region width and thickness of the sample. Thus, phase shift measured by electron holography at 0 V mainly shows the contribution due to the product of V MIP ( x ) and local thickness t ( x ). Under external biases, the term V ext ( x ) describes electrostatic potential distributions due to external biases on the Nb-STO substrate. In a pure dielectric assumption where no mobile charge carriers are considered, application of external bias results in constant electric fields and thus linearly changing electrostatic potentials V ext ( x ) across PZT thin films. However, when there are mobile carriers in the PZT thin film and interface dipoles due to formation of PZT/Nb-STO heterojunction in an electrochemical equilibrium, electric fields due to external biases will be more concentrated around top or bottom interfaces due to corresponding electronic band bending. We extract the changes in electrostatic potential distributions solely caused by external biases ( V ext ( x )) by taking differences between the phase shifts obtained under external bias conditions and that under 0 V as the followings: We estimated the local sample thickness t ( x ) in the reconstructed amplitude images from electron holograms [47] . The sample thickness is found to be linearly increasing towards the substrate ( Supplementary Fig. 2 ). To calibrate thickness from amplitude images, we used 115 nm as the mean free path for inelastic scattering to find thickness profile in Nb-STO region [48] . The determined thickness profile was extended towards the PZT film to obtain whole thickness profile across PZT thin film/Nb-STO substrate to obtain the line profiles of V ext ( x ) using the equation (8). How to cite this article: Han, M.-G. et al . Interface-induced nonswitchable domains in ferroelectric thin films. Nat. Commun. 5:4693 doi: 10.1038/ncomms5693 (2014).